Exceptional river gorge formation from unexceptional floods An understanding of rates and mechanisms of incision and knickpoint retreat in bedrock rivers is fundamental to perceptions of landscape response to external drivers, yet only sparse field data are available. Here we present eye witness accounts and quantitative surveys of rapid, amphitheatre-headed gorge formation in unweathered granite from the overtopping of a rock-cut dam spillway by small-moderate floods ( ∼ 100–1,500 m 3 s −1 ). The amount of erosion demonstrates no relationship with flood magnitude or bedload availability. Instead, structural pattern of the bedrock through faults and joints appears to be the primary control on landscape change. These discontinuities facilitate rapid erosion (>270 m headward retreat; ∼ 100 m incision; and ∼ 160 m widening over 6 years) principally through fluvial plucking and block topple. The example demonstrates the potential for extremely rapid transient bedrock erosion even when rocks are mechanically strong and flood discharges are moderate. These observations are relevant to perceived models of gorge formation and knickpoint retreat. Terrestrial river gorge development within bedrock that exhibits a high unconfined compressive strength (for example, basalt and granite) has implications for understanding similar features on Mars [1] , [2] , [3] , [4] . Numerous studies have examined rates of gorge formation and knickpoint retreat [2] , [5] , [6] , [7] , [8] , [9] , and the controls on those rates via bedrock erodibility [10] , [11] , the effectiveness of mechanisms (bedload abrasion/plucking) [8] , [12] , [13] and the role of hillslope processes [14] . Most findings are based on conceptual and empirical models [11] , [12] , [15] , [16] or long-term landscape analysis, typically using dating techniques and flood reconstruction [5] , [6] , [7] , [17] , [18] . These are plausible approaches but inherently involve unknowns and assumptions. Such issues can be addressed through studies of recent, quantifiable events but examples are scarce and largely restricted to gorges formed in sedimentary rock [17] , [19] , [20] , [21] , [22] , [23] . Quantifying patterns and rates of fluvial erosion into bedrock are essential for understanding linkages between rock strength/structure and discharge, and their influence on landscape evolution [12] . The upstream propagation of steepened reaches in bedrock rivers (that is, knickpoints) is one of the fundamental drivers of landscape evolution, and the rate at which it occurs provides a first approximation to the rate of drainage network response to a base-level change. However, bedrock erosion mechanisms and the rate at which they occur are difficult to establish over long (>10 4 –10 6 year) timescales. While fluvial erosion may appear quasi-continuous, it could conceal long hiatuses that separate incision intervals. This has important implications for the reliability of bedrock river incision as a recorder of external climatic and tectonic forcing [24] . Some studies report contemporary abrupt and episodic fluvial landscape erosion [17] , [19] , [20] , [21] , [22] , [23] . Such studies are rare, yet highly valuable for providing more detailed insights into rates and patterns of fluvial landscape development. Here we present unprecedented evidence for a series of fluvial erosion events that occurred under unremarkable flood discharge conditions over a granite bedrock spillway in the Ricobayo dam (NW Spain). A ∼ 270-m long, ∼ 100-m deep and >100-m wide amphitheatre-headed canyon was carved over 6 years. This case occurred in the early 1930s during the last stages of the dam construction, and represents unique documentation of knickpoint propagation and gorge formation accomplished in a short time interval. This work presents a reconstruction of the evolving stages of river gorge formation by waterfall retreat, integrated with an analysis of the internal and external conditions involved. Together with surprisingly high rates of incision, this example provides evidence of the efficiency of initial bedrock erosion in response to rapid (quasi instantaneous) changes in hydraulic conditions and raises important questions regarding the established models of gorge formation and knickpoint retreat. Dam construction and flood event history The Ricobayo dam was constructed along the Río Esla in NW Iberia in the 1930s. It is located 4-km upstream of the confluence with the Río Duero ( Fig. 1a ), allowing formation of a reservoir (area=57 × 10 6 m 2 , volume=1,150 × 10 6 m 3 ). The Río Esla (287 km in length) has a catchment area of ∼ 16,000 km 2 and a mean (annual) discharge of 5,266 × 10 6 m 3 per year [25] . Before dam construction the Río Esla was characterized by seasonal floods with peak discharges ranging from 500 to >2,500 m 3 s −1 (ref. 26 ), peaking in winter and spring ( Fig. 2a ). Throughout the Ricobayo area the Río Duero and its tributaries have deep gorges ( ∼ 100–450 m) incised into granite and more rarely into metamorphic bedrock [27] . The Ricobayo dam is located in a 100-m deep granite gorge section of the Río Esla. Here bedrock is unweathered but intensely jointed/fractured. The top edge of the granite spillway coincides with a regional low-relief surface ∼ 100 m above the modern Río Esla channel ( Fig. 1c ). 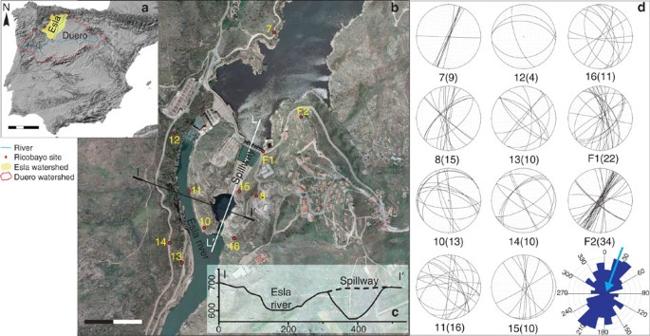Figure 1: Field area and fracture pattern. (a) The Río Esla and Duero watersheds and the study area location. Scale bar, 200-km long; (b) the Ricobayo dam, its spillway and sites of measurements and sampling (orthophotograph, IGN, 2011). Location of longitudinal profile shown inFig. 3iis indicated by L–L′; I–I′ indicates the section shown inc; scale bar, 250-m long (bottom left corner); (c) cross-section showing pre-scour (dashed line) and present topography. (d) Stereoplots of fracture orientations (numbers=location, in brackets the number of fractures plotted). Rose diagram of the whole-fracture population (class interval 15°, maximum percentage 14.6, percentage interval 2%). Arrow shows flow direction of spillway. Figure 1: Field area and fracture pattern. ( a ) The Río Esla and Duero watersheds and the study area location. Scale bar, 200-km long; ( b ) the Ricobayo dam, its spillway and sites of measurements and sampling (orthophotograph, IGN, 2011). Location of longitudinal profile shown in Fig. 3i is indicated by L–L′; I–I′ indicates the section shown in c ; scale bar, 250-m long (bottom left corner); ( c ) cross-section showing pre-scour (dashed line) and present topography. ( d ) Stereoplots of fracture orientations (numbers=location, in brackets the number of fractures plotted). Rose diagram of the whole-fracture population (class interval 15°, maximum percentage 14.6, percentage interval 2%). Arrow shows flow direction of spillway. 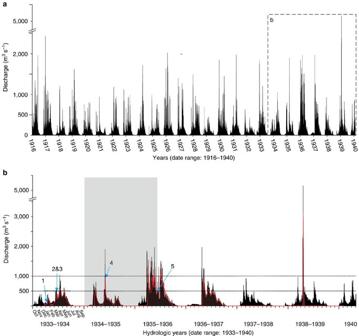Figure 2: Floods entering the reservoir and spillway overtopping discharges. (a) Histogram of the Río Esla water discharge series at Breto Gauging station30,58(1916–1940), which is located upstream of the current dam position close to the current upstream limit of the modern reservoir. (b) Detailed water discharge series (1933–1940 hydrologic years, October–September) showing winter rainfall dominance and scour events. Numbers indicate when main scour events 1–5 occurred. Grey area illustrates the period when spillway lip reinforcements were present. Peak flood discharge in the Río Esla is represented in black and flood discharges exiting the spillway are shown in red. Full size image Figure 2: Floods entering the reservoir and spillway overtopping discharges. ( a ) Histogram of the Río Esla water discharge series at Breto Gauging station [30] , [58] (1916–1940), which is located upstream of the current dam position close to the current upstream limit of the modern reservoir. ( b ) Detailed water discharge series (1933–1940 hydrologic years, October–September) showing winter rainfall dominance and scour events. Numbers indicate when main scour events 1–5 occurred. Grey area illustrates the period when spillway lip reinforcements were present. Peak flood discharge in the Río Esla is represented in black and flood discharges exiting the spillway are shown in red. Full size image The dam and unlined spillway were simultaneously constructed from 1929 to 1933. The reservoir filled with water by the end of 1933 after which a series of spillway overtopping floods occurred [28] characterized by spillway discharges of between ∼ 100 and ∼ 1,500 m 3 s −1 ( Fig. 2b ). These spillway overtopping floods occurred from the middle of December to late June of the 1933–1936 hydrologic years and late January 1936 to the middle of July 1937 ( Fig. 2b ). This led to installation of flood gates at the spillway entrance that increased the reservoir water storage, and evacuation conduits were constructed [29] . After these modifications, only a single but large flood event (a flood of >5,000 m 3 s −1 ) in January 1939 utilized the spillway. The overtopping spillway discharges from this flood (up to 3,000 m 3 s −1 ) exited over a period of 10 days ( Fig. 2b ) [26] , [28] . From January 1934 to March 1936, the flows overtopping the spillway induced scouring that occurred predominantly in five large scour events ( Fig. 3 ). The process was reported by eye witnesses and documented [28] , [29] , [30] . Scour event 1 occurred on 10th January 1934 associated with a spillway discharge of ∼ 80 m 3 s −1 . As a consequence, a 65-m long, 55-m deep gorge was formed ( Fig. 3b,i ). Scour event 2 occurred on 22nd March 1934 associated with a spillway discharge of ∼ 400 m 3 s −1 , producing 75 m of headward erosion and 30–40 m of incision. Further scour (event 3) occurred the next day associated with a ∼ 400 m 3 s −1 spillway discharge, producing a further 100 m of retreat ( Fig. 3c ). The floods continued during April and May and the next winter, but only in 1935 (4th March) during a spillway discharge event of ∼ 1,000 m 3 s −1 was a new large scour (event 4) produced ( Fig. 3d–f ), with an incision of 22 m below the previous erosion level. The last large scour (event 5) occurred in March 1936 (some 500 m 3 s −1 ; Figs 2b and 3g ). Although the erosion occurred predominantly as a result of 5 scour events, minor, intervening erosion from smaller events cannot be ruled out, although eye witness information (survey and photographic data, for example, Figs 3 , 5 and 6 ) suggest these modifications were minor. However, after events 4 and 5, there were several subsequent floods that caused further widening, and block movement at the base of the plunge pool (stage 5 in Fig. 3i ). Thus, we refer to the main scours as ‘events’, and in Fig. 3i refer to ‘stages’ that incorporate both the major event and any minor inter-event modification. 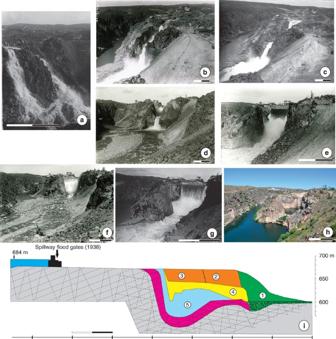Figure 3: Historical imagery looking upstream into the Ricobayo spillway and spillway longitudinal section. Photograph dates: (a) 27/12/1933 before scour event 1; scale bar,∼50-m long; (b) 21/3/1934 after scour event 1; (c) 26/3/1934 2 days after scour event 3; (d) 24/1/1935 scour event 4; (e) 5/3/1935 after scour event 4; (f) 6/7/1935 after scour event 4; (g) 7/4/1936 after scour event 5; (h) 2012. Scale bar,∼100-m long (photographsb–h). (i) Historical long profile sketch of the spillway depict the material removed in each stage (modified from Iberdrola30). Scale bar,∼100-m long. Location is indicated by L–L′ onFig. 1b. Flow from left to right. Successive erosion stages (represented by different colours) include the main scour events (1–5) and minor inter-event scouring. Pink area indicates the bedrock reinforced during the concrete revetment work post gorge formation (1940s onwards,h). Spillway flood gates represented were installed in 1938. (Imagery credit Iberdrola). Figure 3: Historical imagery looking upstream into the Ricobayo spillway and spillway longitudinal section. Photograph dates: ( a ) 27/12/1933 before scour event 1; scale bar, ∼ 50-m long; ( b ) 21/3/1934 after scour event 1; ( c ) 26/3/1934 2 days after scour event 3; ( d ) 24/1/1935 scour event 4; ( e ) 5/3/1935 after scour event 4; ( f ) 6/7/1935 after scour event 4; ( g ) 7/4/1936 after scour event 5; ( h ) 2012. Scale bar, ∼ 100-m long (photographs b – h ). ( i ) Historical long profile sketch of the spillway depict the material removed in each stage (modified from Iberdrola [30] ). Scale bar, ∼ 100-m long. Location is indicated by L–L′ on Fig. 1b . Flow from left to right. Successive erosion stages (represented by different colours) include the main scour events (1–5) and minor inter-event scouring. Pink area indicates the bedrock reinforced during the concrete revetment work post gorge formation (1940s onwards, h ). Spillway flood gates represented were installed in 1938. (Imagery credit Iberdrola). Full size image Figure 5: Contour maps of the spillway topography showing the erosion sequence. 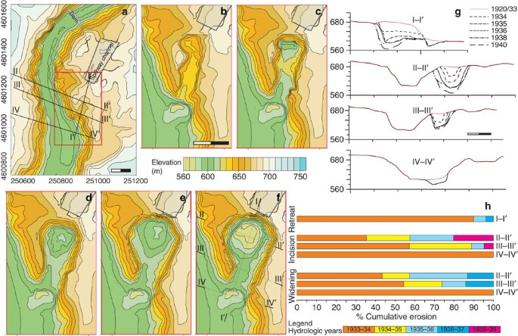Figure 5: Contour maps of the spillway topography showing the erosion sequence. Contour lines=10-m intervals. Map dates: (a) 1920; box=area represented inb–f; Dam and present location of the spillway channel represented. (b) 1934 (after scour events 1–3); (c) 1935 (after scour event 4); (d) 1936 (after scour event 5); (e) 1938; (f) 1940; (g) sections of spillway site in successive years (seeafor location). Scale bar, 100-m long. (h) Plot of cumulative percentage of retreat, incision and widening along different gorge sections. Upper reach (II–II′), middle reach (III–III′) and lower reach (IV–IV′). Contour lines=10-m intervals. Map dates: ( a ) 1920; box=area represented in b – f ; Dam and present location of the spillway channel represented. ( b ) 1934 (after scour events 1–3); ( c ) 1935 (after scour event 4); ( d ) 1936 (after scour event 5); ( e ) 1938; ( f ) 1940; ( g ) sections of spillway site in successive years (see a for location). Scale bar, 100-m long. ( h ) Plot of cumulative percentage of retreat, incision and widening along different gorge sections. Upper reach (II–II′), middle reach (III–III′) and lower reach (IV–IV′). Full size image Figure 6: Spillway erosion pattern and erosion rates. 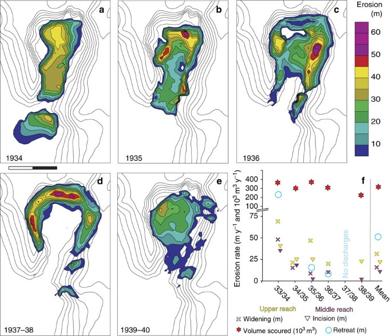Figure 6: Spillway erosion pattern and erosion rates. (a–e) Contour maps of erosion (spillway surface lowering) that occurred during a series of scour events (1934–1940). Contour interval=10 m. Scale bar, 100-m long. Bottom left dates indicate the years when the topographic surveys were performed. (a–c) Maps represent a 1-year period; (d,e) maps correspond to 2-year intervals. (f) Plot of erosion that occurred in the spillway for successive years (1933–1939). Erosion values obtained through DEM reconstruction and measured along selected sections (Methods) illustrate the evolution of the upper and middle reaches (yellow and purple symbols, sections II–II′ and III–III′, respectively, inFig. 5). Mean erosion values (retreat, incision, widening and eroded volume) are total erosion over the years when discharges occurred (that is, 5 years, as there were no spillway discharges in 1937–1938 hydrologic year—seeFig. 7). Where data for the same year are presented (for example, 35/36) symbols for the upper and middle reaches are represented with a small horizontal offset to facilitate visualization. ( a – e ) Contour maps of erosion (spillway surface lowering) that occurred during a series of scour events (1934–1940). Contour interval=10 m. Scale bar, 100-m long. Bottom left dates indicate the years when the topographic surveys were performed. ( a – c ) Maps represent a 1-year period; ( d , e ) maps correspond to 2-year intervals. ( f ) Plot of erosion that occurred in the spillway for successive years (1933–1939). Erosion values obtained through DEM reconstruction and measured along selected sections (Methods) illustrate the evolution of the upper and middle reaches (yellow and purple symbols, sections II–II′ and III–III′, respectively, in Fig. 5 ). Mean erosion values (retreat, incision, widening and eroded volume) are total erosion over the years when discharges occurred (that is, 5 years, as there were no spillway discharges in 1937–1938 hydrologic year—see Fig. 7 ). Where data for the same year are presented (for example, 35/36) symbols for the upper and middle reaches are represented with a small horizontal offset to facilitate visualization. Full size image During the time periods following the scour events, some engineering work was attempted in the spillway to mitigate the scouring. By the summer of 1934 this had involved localized concrete sealing of the spillway channel and concrete reinforcement of the spillway lip. In 1935, concrete patches were built at selected points in the plunge pool to avoid further block movements, and a small ramp and an overhanging lip were constructed at the spillway crest. However, concrete reinforcements were systematically damaged during subsequent overtopping events with almost complete removal by floods in March 1936, including the reinforcements in the spillway lip [28] . The situation was finally ‘controlled’ when hydraulic splitters were added (post 1940) to the end of the spillway channel to break up the jet of the overtopping flood water before it entering the plunge pool [28] . Bedrock material properties Field work was designed to examine bedrock erodibility and structural discontinuity patterns (fractures, fault and joint planes) of the local geology. Rock strength measurements utilized a Schmidt hammer [31] , [32] for in situ field testing, and a laboratory slake durability test [33] on rock samples to provide information on the mechanical strength and erodability of the bedrock (Methods). Schmidt hammer analyses were performed in the Ricobayo dam area and the downstream Río Duero gorge ( Supplementary Table 1 ). Measurements targeted areas of potentially different weathering histories (that is, scour site, natural Río Esla gorge wall, dam quarries, road cuts, tunnel, natural outcrops, fault planes and a single highly weathered surface site) from surface locations ( Fig. 1b ) and down to ∼ 80 m below the surface within a dam tunnel (site 12, Fig. 1b ). Average Rebound ( R ) values ranged from 17 to 44. Lower values (<30) corresponded to surfaces with longer-term weathering histories, while higher values (34–44) corresponded to unweathered outcrops (for example, tunnel R =43). The relationship of R values to weathering history was concordant between Ricobayo and the downstream Río Duero gorge area ( Supplementary Table 1 ). The slake durability test [33] was applied to samples collected from Schmidt hammer measurement sites ( Supplementary Table 1 ). Durability index values were systematically >95, with the unweathered bedrock possessing a ‘very high durability’ at both Ricobayo and in the downstream Río Duero gorge. Bedrock discontinuities Systematic measurements of fractures (joints and faults, see Methods) revealed a pattern in the Ricobayo area dominated by NNE–SSW striking fractures ( Fig. 1d ). This included a primary NNE left-lateral strike-slip fault system concordant with previous field-based regional structural geological analyses [34] , [35] . This primary pattern exerts a significant control on drainage network orientation, as observed in the lower Río Esla reach ( Supplementary Fig. 1 ). Secondary fracture sets oriented NNW-SSE and ESE-WNW are encountered and are significant at outcrop scale ( Figs 1d and 4 ). Most fractures were vertical or near-vertical, although minor subhorizontal unloading joints were also present. Fracture spacing was locally in a 0.3–3 m range ( Supplementary Table 1 ) and fracture length is typically more than several tens of metres, with a vertical persistence along the whole outcrop ( Fig. 4 ). Exposures of discontinuity surfaces revealed a dominance of fresh, tight and unweathered planes. Fracture plots suggest that the primary fracture sets influence river incision and the progression of erosion in the spillway. 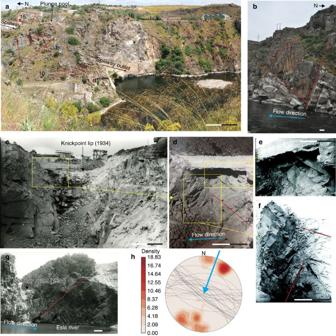Vertical and sub-vertical NNW to NNE trending structures determine the bedrock river and spillway gorge orientation (for example, site 15 in Figs 1 and 4a ). ESE trending fractures are orthogonal to flow direction in the spillway with sets dipping both against and towards the flow ( Figs 1d and 4 ). Figure 4: Field photographs illustrating fracture geometry at the spillway site and Río Esla. (a) Present spillway outlet and fracture pattern. Red dots indicate measurement sites (Fig. 1), red lines indicate fracture planes. Red box at site 15 represents a∼N–S fault plane outcrop, parallel to the spillway gorge orientation. Scale bar,∼50-m long. (b) Western side of the Río Esla in front of site 11 (Fig. 1b). Fracture set dipping against and toward the flow. Scale bar,∼1-m long. (c) Spillway lip and gorge formed during 1933–1934 hydrologic year (scours 1–3;Fig. 3); scale bar,∼50-m long, (credit Iberdrola). Yellow box indicates location of photographd. (d) Fracture pattern at the knickpoint lip by summer 1934 when retreat had significantly slowed (credit Iberdrola). Scale bar,∼25-m long; Yellow boxes indicate location of photographs (e,f). (e) Detail of fracture orientation (dipping against the flow) at the knickpoint lip. Scale bar,∼25-m long. (f) Detail of fracture orientation (dipping predominantly toward the flow) downstream of the knickpoint lip. Scale bar,∼25-m long; (g) Fracture sets dipping predominantly against the flow at the∼30-m height knickpoint formed at the spillway outlet (confluence with the Río Esla) by March 1934. This knickpoint disappeared during the fourth main scour (Fig. 3d,e) in March 1935. Scale bar, 25 m. (h) Orthogonal to flow fracture planes dipping towards and against the flow. Stereoplot and density plot of ESE trending fractures, measured at the Ricobayo sites (see Methods). Figure 4: Field photographs illustrating fracture geometry at the spillway site and Río Esla. ( a ) Present spillway outlet and fracture pattern. Red dots indicate measurement sites ( Fig. 1 ), red lines indicate fracture planes. Red box at site 15 represents a ∼ N–S fault plane outcrop, parallel to the spillway gorge orientation. Scale bar, ∼ 50-m long. ( b ) Western side of the Río Esla in front of site 11 ( Fig. 1b ). Fracture set dipping against and toward the flow. Scale bar, ∼ 1-m long. ( c ) Spillway lip and gorge formed during 1933–1934 hydrologic year (scours 1–3; Fig. 3 ); scale bar, ∼ 50-m long, (credit Iberdrola). Yellow box indicates location of photograph d . ( d ) Fracture pattern at the knickpoint lip by summer 1934 when retreat had significantly slowed (credit Iberdrola). Scale bar, ∼ 25-m long; Yellow boxes indicate location of photographs ( e , f ). ( e ) Detail of fracture orientation (dipping against the flow) at the knickpoint lip. Scale bar, ∼ 25-m long. ( f ) Detail of fracture orientation (dipping predominantly toward the flow) downstream of the knickpoint lip. Scale bar, ∼ 25-m long; ( g ) Fracture sets dipping predominantly against the flow at the ∼ 30-m height knickpoint formed at the spillway outlet (confluence with the Río Esla) by March 1934. This knickpoint disappeared during the fourth main scour ( Fig. 3d,e ) in March 1935. Scale bar, 25 m. ( h ) Orthogonal to flow fracture planes dipping towards and against the flow. Stereoplot and density plot of ESE trending fractures, measured at the Ricobayo sites (see Methods). Full size image Bedrock erosion Reconstruction of the scour site topography before the dam construction (1920) and for successive years during the erosion events (1934–1940) was performed through analysis of historic topographic maps [28] , [29] (Methods). Digital elevation model (DEM) generation illustrates the former topography of the spillway site and how the bedrock erosion proceeded ( Fig. 5 ). Comparison of successive DEMs enabled spatial and temporal erosion patterns to be quantified for successive stages and allows the calculation of erosion rates (incision, widening, retreat and eroded volume; Fig. 6 ). Before the erosion events dam workers established a low gradient (<1°) unlined rock spillway channel. The channel, 400-m long, was inset ∼ 20 m into the bedrock on a topographic high ( ∼ 70 m above the riverbed; Figs 3i and 5a ). The downstream boundary of the spillway was formed by a high angle ( ∼ 30°) knickpoint lip perpendicular to flow that had been artificially created in the spillway mouth ( Figs 3 and 5a,g ). By the summer of 1934 scour events had formed a 230-m long, 35-m deep and 90-m wide bedrock canyon, excavating a 20-m deep plunge pool in the Esla riverbed at the spillway outlet and achieving ∼ 90% of the overall gorge headward erosion ( Figs 5b,g,h and 7 ). Collectively, 369,300 m 3 of rock was removed ( Fig. 6a,f ). The 1935 map ( Fig. 5c ) shows the spillway topography after the fourth large scour event. In 1 year, overtopping discharges created widening (20±2 m) and incision (20-m mean) along the previous canyon ( Fig. 6f ), with localized incision (>50 m) in the newly formed plunge pool ( Figs 5g and 6b ). By this time, the middle reach had accomplished almost 90% of its total incision, while the upper reach had accomplished <60% ( Fig. 5h ). The volume of rock removed was 302,561 m 3 . From late 1935–1937, most of the gorge widening ( ∼ 70 m, Fig. 6f ) took place in the upper reach, leading to the development of an amphitheatre-headed valley ( Fig. 5d,e ). During this period, the maximum incision (>50 m) occurred along the uppermost external edge of the gorge producing headwall retreat of ∼ 30 m (mean) ( Fig. 6c,d ) and thus the destruction of the spillway lip reinforcements (March 1936). This is a stage where headward erosion and widening dominated ( Fig. 6c,d,f ). The volume of rock removed during this phase was 687,857 m 3 . After late July 1937 no discharges were evacuated though the spillway with the exception of the January 1939 event previously described ( Fig. 2b ), during which erosion was focussed in the floor of the amphitheatre ( Figs 5f and 6e ), achieving 20% of the total incision in the upper reach ( Fig. 5h ) and removing a volume of 221,495 m 3 . Thus, a ∼ 270-m long, ∼ 100-m deep and ∼ 100–160-m wide canyon was carved over 6 years, and ∼ 1.58 × 10 6 m 3 of granite bedrock was removed from the spillway site and mostly deposited downstream along the Esla riverbed (see images in Fig. 3 ). The cumulative percentage of incision, widening and headcut over time exhibit different step patterns indicating the episodic nature of the erosional process ( Figs 5h and 7 ). Moreover, the spatial analysis of erosion along different sections of the canyon illustrates how erosion migrates with headwall retreat ( Fig. 5g,h ). For the studied period, 100% of erosion is achieved during the first hydrologic year in the lower reach, while in the middle and upper reaches incision and widening is sustained over a further 3–4 hydrologic years. Thus, the gorge progressively changed shape, initially dominated by headward retreat, then widening and vertical incision into the existing amphitheatre-headed gorge ( Figs 6 and 7 ). 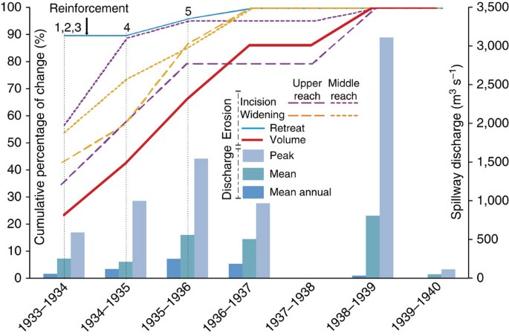Figure 7: Plots of spillway gorge erosion and spillway flood discharges by hydrologic year. Numbers on chart area indicate the scour events (1–5). Erosion values are those obtained by DEM reconstruction (Figs 5and6) per hydrologic year. Cumulative percentage plot of volume eroded, retreat (measured along section I–I′ inFig. 5), and incision and widening measured in the upper and middle reaches (sections II–II′ and III–III′, respectively, inFig. 5). Mean discharge is calculated as the total spillway discharge during a hydrologic year averaged over the overtopping period. Mean annual discharge is calculated as the total spillway discharge averaged over a hydrologic year. Peak discharge is the maximum spillway overtopping flood occurring during the hydrologic year. Figure 7: Plots of spillway gorge erosion and spillway flood discharges by hydrologic year. Numbers on chart area indicate the scour events (1–5). Erosion values are those obtained by DEM reconstruction ( Figs 5 and 6 ) per hydrologic year. Cumulative percentage plot of volume eroded, retreat (measured along section I–I′ in Fig. 5 ), and incision and widening measured in the upper and middle reaches (sections II–II′ and III–III′, respectively, in Fig. 5 ). Mean discharge is calculated as the total spillway discharge during a hydrologic year averaged over the overtopping period. Mean annual discharge is calculated as the total spillway discharge averaged over a hydrologic year. Peak discharge is the maximum spillway overtopping flood occurring during the hydrologic year. Full size image The dominance of tight and unweathered fracture planes, together with the rock strength analyses show that the Ricobayo granite is mechanically strong. The local spillway strength data ( Supplementary Fig. 1 ) demonstrate that bedrock here is no weaker than elsewhere, since similar rock strength and fracture patterns are found in the regional geological context. However, discontinuity patterns through fracture density and orientation interactions play an important role in the gorge development [12] , [20] , [36] . The existence of several fracture sets with different orientations resulted in the formation of bedrock blocks that were susceptible to removal by plucking and probable block topple ( Fig. 4 ). Similar (m-scale) blocks can be found elsewhere in the natural reaches of the Río Esla suggesting this is not just localized to the spillway area. The NNW to NNE structures regionally determines channel orientation patterns. Furthermore, although they are quantitatively less represented, the orthogonal to flow fracture sets within these channels play a key role in the gorge progression. This structural pattern ( Fig. 4 ) enhances headward erosion when the fractures dipped towards flow and favoured incision when fractures dipped predominantly against flow [20] , [36] . Knickpoint upstream propagation was extremely rapid (>230 m per y) during the first stages of the gorge formation (main scours 1–3; Fig. 3 ), but decreased rapidly thereafter ( Fig. 6f ), superseded by incision and gorge widening ( Figs 5 , 6 , 7 ). The knickpoint lip reinforcement attempts made in summer 1934 could have some influence on this pronounced slowdown in knickpoint retreat, acting in the manner of a resistant cap rock [37] . Observations and flow data ( Figs 2b , 3 and 4 ), however, suggest otherwise. Between scour event 3 (spring 1934) and the introduction of the artificial reinforcement (summer 1934) there were several spillway overtopping discharges that were similar or higher in magnitude to the events that created the initial gorge ( Fig. 2b ) but these spillway floods did not cause knickpoint retreat. This would imply that the pronounced decrease in headward retreat rates had already occurred before the introduction of the artificial reinforcement ( Fig. 7 ). Furthermore, the knickpoint reinforcements were only a temporary feature as they were ripped out by flooding in March 1936. While waterfall lip shape, length and height are thought to be influential in affecting waterfall retreat rates [38] , other studies have highlighted bedrock structure and fracture geometry as playing a fundamental role in block stability [36] , [39] , knickpoint morphology and retreat rate [6] , [11] , [20] , [40] . In this example, the slowdown in retreat rate appears to mirror the timing of when the knickpoint interacts spatially with the area dominated by anti-flow oriented fracture sets, implying that that structural differences along the gorge, with local predominance of fracture sets dipping against the flow, became significant in suppressing the retreat progression [30] ( Fig. 4d–g ). During the initial stage of spillway operation, the jet produced by the ∼ 70 m waterfall at the confluence of the spillway channel with the Río Esla, created the lower plunge pool at the riverbed ( Figs 5b and 6a ). Rapid modification of the spillway bed morphology by episodic, predominantly headwall retreat during the ensuing gorge creation ensured that this initial knickpoint was only temporary (months) and thus the lower plunge pool was limited in extent. As the headward retreat slowed (1934), a new near-vertical face ( ∼ 30-m height, Fig. 4c ) was formed at the spillway channel outlet, 230-m upstream. The position of this knickpoint was fixed in place over a relatively longer timescale (years), thus having the opportunity to develop a more pronounced, upper plunge pool feature. During the following hydrologic year, this upper headwall significantly increased in height, by scouring (March 1935), while the former waterfall that had existed at the confluence was almost completely erosionally removed ( Figs 3 and 5 ). Under this latter configuration the lower plunge pool that initially formed in the lower reach (sections IV–IV′, Fig. 5 ) progressed no further ( Fig. 6 ), but instead a new (upper) plunge pool was initiated in the upper reach, at the base of the active headwall (sections II–II′ in Fig. 5 ). During subsequent overtopping periods, the upper plunge pool was developed, initially by the water jet impact over the knickpoint directly onto the riverbed. Thereafter, as the water depth increased in the plunge pool with successive outflow discharges and progressive scour formation, the water jet energy focused on the developing plunge pool water body [41] , [42] . Over this time bedrock scours occurred predominately at the base of the plunge pool and incision in the middle reach was minimal ( Figs 5g,h and 6 ). Subsequently, as the channel was deepened and enlarged, the rim of the headwall and the gorge sides became unstable and the canyon began widening. Thus, while headwall retreat moved as a wave of erosion upstream creating the canyon, the slowdown in retreat rate promoted a persistent vertical headwall, allowing incision and widening to progress ( Fig. 7 ) and eventually forming the present amphitheatre-headed valley with a 40 m water depth plunge pool ( Figs 5 and 6 ). During the rapid phase of gorge formation, abrasion was considered to be minimal as the river sediment load would have been largely entrapped within the reservoir behind the dam. Although negligible, some erosion by abrasion may have occurred within the plunge pool associated with dislodgement and transport of the scoured blocks from the plunge pool [13] , [43] , [44] . None of the existing documentation or photographs observed within the archives suggests any evidence to support spring seepage as an active process at any stage of erosion. Given the bedrock strength and short time period, it is considered that if this process was at all active it would be of minimal impact [1] . Thus, the dominant erosional processes must relate to surface water flow and the scour must be explained by physical–mechanical processes relating to surface water discharge and its interaction with the underlying bedrock [40] , [45] . Given the morphology of the spillway channel and structural pattern of the bedrock, the most likely mechanisms are hydraulic jacking of the rock mass, causing a progressive break-up of rock fractures due to fluctuating pressures; with dynamic extraction of single rock blocks and downstream displacement and/or deposition of the broken-up material. According to this model, between any two successive large scour events the erosional threshold for block plucking must have been attained [40] . In this example, the scours appear as discrete events despite the continuity of floods that occurred between them ( Fig. 2b ). Peak and mean discharges display no relationship with volume of bedrock eroded ( Fig. 7 ). Thus, the most plausible explanation for the discontinuous erosion pattern is that incision rate is limited by hydrodynamic joint-block extraction [12] . Before and during dam construction, much larger floods (up to 2,500 m 3 s −1 ) occurred in the Río Esla ( Fig. 2 ) [26] , [46] but they were not associated with any significant erosion within the spillway gorge. The elevated stream power caused by the artificially created waterfall in the ‘spillway channel’ outlet is suggested as the driving mechanism for rapid knickpoint retreat and gorge formation. This example demonstrates retreat, incision and widening rates of 10–10 2 m per year ( Fig. 6f ). In comparison with worldwide data [2] , [47] both the long-term and short-term knickpoint recession rates of this example are extremely high. Even when compared with the biggest waterfalls in the world, retreat rates observed at Ricobayo are orders of magnitude higher (1.2–2 m per year for Niagara [37] and >0.15 m per year Victoria [48] Falls). However, when compared with existing rare eye witness examples of a sudden disequilibrium that affects a river system, for example, drainage diversion [21] , [22] , extraordinary flood [17] , differential uplift along the riverbed [20] , [23] or dam removal [49] similar rates of the river adjustment to new conditions (incision, retreat and widening) are found. Such data imply that the response of bedrock rivers to external environmental perturbations, even in mechanically strong rock, can be extremely rapid in the initial stages, and episodic rather than quasi-continuous. Long-term landscape erosion rates generally tend to be orders of magnitude smaller as these initial rapid phases of adjustment are concealed by relative hiatuses in erosional activity over longer time periods [24] . Overall, this study highlights several key observations concerning the morphological adjustment of bedrock rivers on Earth and Mars [50] , [51] , [52] that are particularly pertinent in the study of geomorphological phenomena such as extreme flood discharge events and river diversions through drainage capture and overspill: (1) that moderate water discharges (<1,500 m 3 s −1 , in this example) are capable of radical erosion suggesting that adjustments to changes such as drainage diversion and capture may be initially much more rapid than has hereto been assumed [53] , [54] ; (2) that megafloods are not a prerequisite for major erosion events in mechanically strong lithologies; (3) that such radical erosion is strongly facilitated by a favourable discontinuity pattern in mechanically strong rocks even in the absence of significant surface weathering, and that this discontinuity pattern also strongly influences the gorge morphology; (4) that the key removal process in such rocks would appear to be fluvial plucking probably in association with block topple; (5) that spring sapping is not essential to develop an amphitheatre-headed gorge in resistant bedrock lithologies [1] , [4] ; and (6) that extreme erosion rates are possible even in the absence of bedload and suspended load. Furthermore, these observations have implications for the efficiency of bedrock erosion and raise important questions about incision rates, driving mechanisms and timescale assumptions for models of landscape evolution over a variety of temporal and spatial scales and for modern engineering strategies. Schmidt hammer An N-type Schmidt hammer was used following procedures outlined by [31] , [32] . At each site, 32 horizontal hammer impacts were taken from the exposed rock surface. The maximum and minimum values were considered as outliers and were excluded from the data set, with mean R values calculated from the remaining 30 measurements. Schmidt hammer measurements were obtained from 16 outcrops along the Río Duero gorge, in the Ricobayo spillway and its nearby area ( Supplementary Fig. 1 ). Measurements were taken from an unweathered tunnel, with the remaining 15 outcrops representing varying degrees of natural weathering in road cuts, quarries and river gorges. These include strongly weathered outcrops, asociated with long-term surface exposure (site 1) or highly weathered fault planes (sites 6 and 8), and sites with relatively fresh rock outcrops. Slake durability test and durability index The slake durability test [33] is regarded as a simple test for assessing the influence of weathering on rock and its ability to resist abrasion and breakdown. It estimates the resistance of rock to a combination of wetting and abrasion cycles based on ASTM D4644-87 (ref. 55 ). The test provides a durability index of a rock after two drying and wetting cycles with abrasion. For each test, 10 representative, intact, roughly equidimensional fragments of rock, each of mass 40–60 g, are placed in a wire-mesh drum (2 mm), which is partially immersed in water and rotated at 20 r.p.m. for 10 min. As the fragments disintegrate, the fine fractions pass through the mesh. Each group of samples was subjected to two cycles. The samples are oven-dried and weighed before and after each cycle. The durability index is an expression of the average dry weight percentage of rock retained in the testing drum after each cycle. High durability=95–98% retention and very high durability≥98% retention [33] , [56] . The slake durability test was used as a comparison between the spillway bedrock and that exposed throughout the study area. Nine sites were examined to encompass subtle granite lithological variations and weathering variabilities ( Supplementary Fig. 1 ; Supplementary Table 1 ). Fracture population analysis Field survey was undertaken to identify the bedrock fracture pattern. Orientation (trend and dip) of 151 fracture (fault and joint) planes were measured at 11 sites in the Ricobayo area ( Fig. 1d ). This task was preceded by field reconnaissance to select representative outcrops that encapsulated all of the fracture types and patterns. Stereoplots, histograms, rose diagrams and density plots were used to analyse the data. The fracture pattern is dominated by NNE–SSW striking structures, while secondary fracture sets oriented NNW-SSE and ESE-WNW take weight at outcrop scale ( Fig. 1d ). Together with the statistical analysis, the dominant trends were identified from aerial and field imagery and then compared with published regional fault patterns [34] ( Supplementary Fig. 1 ). Due to the relevance of dip and dip direction of the ortogonal to flow fracture sets in the erosional process [36] , [57] and based on field experience ( Fig. 4a–d ), ESE trending sets were analysed separately. Planes striking within N85° E and N140° E were extracted from the whole population and represented by a stereoplot and density diagram ( Fig. 4h ). DEMs and erosion quantification DEMs of the spillway area were constructed from digitized and georeferenced topographic maps before dam constrution (1920) and during the scour events (1934–1940). Historical topographic maps used to derive the DEMs were originally drawn at 1:1,000 scale with a 5-m countour interval. These historical DEMs were compared with the modern 5 m DEM from the Instituto Geográfico Nacional, allowing interpolation and the construction of 5-m DEMs and countour maps for successive scour events ( Fig. 5 ). The surveys for the compilation of the historical contour maps were conducted during dry periods (summer months). Thus, the resultant interpolation maps represent gorge and plunge pool geometries of successive years. In some instances, these periods spanned several main scour events. To quantitatively illustrate how erosion evolves in different sections of the gorge (longitudinally and in the upper, medium and lower reaches), retreat, incision and widening occurred in successive hydrologic years was measured along selected sections (I–I′ to IV–IV′, in Fig. 5 ). Cumulative percentages of erosion along these sections are illustrated in Fig. 5h . The geometry and volume of the gorge produced by successive scour events were calculated through subtraction of DEM topography of consecutive years. The resulting contour erosion maps for successive periods are shown in Fig. 6 . How to cite this article: Anton, L. et al. Exceptional river gorge formation from unexceptional floods. Nat. Commun. 6:7963 doi: 10.1038/ncomms8963 (2015).